A rational design of cosolvent exfoliation of layered materials by directly probing liquid–solid interaction Exfoliation of layered materials such as graphite and transition metal dichalcogenides into mono- or few-layers is of significant interest for both the fundamental studies and potential applications. Here we report a systematic investigation of the fundamental factors governing the liquid exfoliation process and the rational design of a cosolvent approach for the exfoliation of layered materials. We show that Young’s equation can be used to predict the optimal cosolvent concentration for the effective exfoliation of graphite and molybdenum disulphide in water mixtures with methanol, ethanol, isopropanol and t-butyl alcohol. Moreover, we find that the cosolvent molecular size has an important role in the exfoliation yield, attributed to the larger steric repulsion provided by the larger cosolvent molecules. Our study provides critical insight into the exfoliation of layered materials, and defines a rational strategy for the design of an environmentally friendly pathway to the high yield exfoliation of layered materials. Two-dimensional layered materials (LMs) are characterized by their strong in-plane bonds and weak van der Waals (vdW)-like coupling between the layers. With the discovery of graphene, there has been a growing interest in single or few-layers of exfoliated LMs. These materials can form a natural two-dimensional crystal structure and offer promising opportunities for both fundamental studies and technological applications. Graphene has been explored for a wide variety of uses, such as transparent conductors, transistors and biological sensors [1] , [2] , [3] , [4] . Transition metal dichalcogenides such as molybdenum disulphide (MoS 2 ) and tungsten disulphide are semiconducting and have shown significant potential for use in electronic devices, energy storage and catalytic purposes [5] , [6] , [7] . Other transition metal dichalcogenides such as niobium diselenide (NbSe 2 ) are metallic, and have been shown to be superconducting at low temperatures [8] . While the bulk syntheses of these materials have been successful, ways of producing large-scale mono/few-layers are still limited. Currently, the highest yielding exfoliation process from a bulk starting material is restricted to chemical modification through intercalation, oxidation or functionalization [9] , [10] , [11] , [12] , [13] , [14] . However, the chemical reactions involved in the aforementioned processes can often introduce a large number of defects or dopants to the crystal structure and severely alter or degrade the intrinsic properties of the resulting materials [9] , [10] , [11] , [12] , [13] , [14] , [15] , [16] . Exfoliation methods without a chemical reaction are preferred in order to maintain the structural and electronic integrity of the material. Recent studies have shown that LMs can be directly exfoliated by sonication in a properly selected solvent [17] , [18] , [19] , [20] , [21] . If the yield can be improved, the solvent exfoliation method is largely preferred because, unlike the common lithium intercalation method, liquid exfoliation is not an air-sensitive process and does not involve chemical reactions. These factors improve the processability while maintaining the intrinsic properties of LMs. However, there is not yet a good method to evaluate the suitability of a solvent for the effective exfoliation of LMs. The exploration of this subject is largely being developed through a trial-and-error process by testing a large number of solvents. So far, N -methyl-2-pyrrolidone (NMP) and other pyrrolidone-based solvents are found to be the more effective exfoliating solvents for both graphite and MoS 2 (refs 17 , 18 ). However, these pyrrolidone-based solvents are generally toxic and have a high-boiling point. Classified as a reproductive toxin, industrial scale use of such solvent may pose a significant environmental risk [22] , [23] . On the other hand, it has been demonstrated that drugs and polymers show a cosolvency effect in which the solubility of a material can be greatly improved by using a mixture of solvents while showing low or no solubility in either of the individual components of the mixture [24] , [25] , [26] , [27] . Demonstrated by the isolation of monolayers of graphene and MoS 2 with scotch tape [1] , [7] , [28] , the basal plane of both graphite and MoS 2 displays a strong vdW-like interaction. The nature of plane-plane vdW-like interaction of LMs is fundamentally similar enough to that of polymers. Given the right solvent mixture, similar cosolvency effect observed in polymer materials can also occur in these LMs [20] , [21] . Indeed, it has been recently shown that LMs can be exfoliated using a mixture solvent of water and ethanol (ETA) [21] . To rationalize the experimental data observed, recent studies have used the Hansen solubility parameters (HSP) as an explanation [17] , [18] , [21] . The HSP works by assigning values on the extent of a materials’ ability to form dispersion, polar and H-bonding interactions (H-bond does not mean exclusively hydrogen bonding, but rather everything else not accounted for by dispersion and polar). The HSP of a material are extracted by testing its solubility in a large number of solvents of known solubility parameters and finding the best fit [29] . However, it is usually a challenge to obtain all three solubility parameters due to the large test pool needed. In addition, the HSP intrinsically assumes that solvents only engage in three distinct interactions, and neglect other possible interactions. As a result, it can causes uncertainty that makes it difficult to determine the best exfoliation solvent in a predictable manner. Here we explore the fundamental factors governing the liquid exfoliation process through a rational design of a cosolvency approach for the exfoliation of graphite and MoS 2 in a simple water–alcohol mixture. We demonstrate by directly determining the liquid–solid interfacial energy through contact angle measurement, it is possible to predict the optimal cosolvent concentrations for the effective exfoliation of LMs without the need to make any assumption on the material’s solubility parameters or the exact nature of the material–solvent interactions. Moreover, we find that molecular size of the cosolvent system can have an important role in the exfoliation yield. Solvent–solid interaction Equilibrium contact angle of water–solvent mixture was measured on highly ordered pyrolytic graphite (HOPG) and large MoS 2 single crystals. As an experimental control, we chose methanol (MET), ethanol (ETA), isopropanol (IPA), and t-butyl alcohol (TBA) as cosolvents. These solvents were chosen because their chemical structures differ only by the substitution of –H group with –CH 3 bounded to the central carbon atom. Owing to the similar nature of the alcohols, we expect that a greater clarity in exfoliation trends would emerge through the use of these selected solvents rather than through the use of a wide range of randomly chosen solvents. To predict thermodynamic stability, we used Young’s Equation by evaluating the change in interfacial energy [30] , [31] : where γ sl, γ sg and γ lg are the solid–liquid, solid–gas, and liquid–gas interfacial energy, respectively, and θ c is the equilibrium contact angle. For a liquid, γ lg is equal to its surface tension, and its value is usually well known from published sources or can be measured by using a goniometer [32] , [33] . γ sg represents interfacial energy between solid and atmosphere and does not change regardless of the solvent used, it therefore simply acts as a constant in the equation and can be readily subtracted out of the equation when comparing two different solvents. This is beneficial because the γ sg value varies substantially for graphite in literature (100–200 mJ m −2 ) (refs 34 , 35 ) and is largely unreported for MoS 2 . Calculating the solid–liquid interfacial energy ( γ sl ) directly would produce large uncertainty. Thermodynamically, the most stable interaction should occur when the value of γ sl is minimized or, equivalently, when γ lg cos θ c is maximized when considering γ sg as a constant for a given LMs. Therefore, when comparing the interfacial energy between a given LM with two different solvents, the only factors needed are the surface tension of the solvent ( γ lg ) and the solid–liquid contact angle ( θ c ). Both of these parameters can be readily measured experimentally for any solvent system ( Fig. 1a–d ). Therefore, this approach can be used for evaluating essentially an arbitrary solvent mixture. 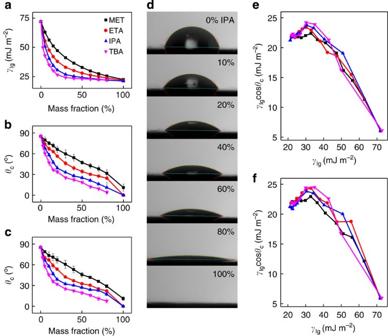Figure 1: Probing minimum solid–liquid interface energy. (a) Surface tension of water–alcohol mixture at various weight fraction at 25 °C (refs32,33). Tested solvents: MET (black squares), ETA (red circles), IPA (blue triangles), TBA (purple inverted triangles). (b,c) Contact angles of various cosolvents (water-alcohols) on HOPG (b) and MoS2(c). (d) Photographs of contact angle measurements of water–IPA cosolvent system at various concentrations on graphite. (e,f) The calculated decrease in solid–liquid interfacial energy (γlgcosθc) based on Young’s equation shows a thermodynamic minimum occurring at surface tension of 30–35 mJ m−2for both HOPG (e) and MoS2(f). Figure 1: Probing minimum solid–liquid interface energy. ( a ) Surface tension of water–alcohol mixture at various weight fraction at 25 °C (refs 32 , 33 ). Tested solvents: MET (black squares), ETA (red circles), IPA (blue triangles), TBA (purple inverted triangles). ( b , c ) Contact angles of various cosolvents (water-alcohols) on HOPG ( b ) and MoS 2 ( c ). ( d ) Photographs of contact angle measurements of water–IPA cosolvent system at various concentrations on graphite. ( e , f ) The calculated decrease in solid–liquid interfacial energy ( γ lg cos θ c ) based on Young’s equation shows a thermodynamic minimum occurring at surface tension of 30–35 mJ m −2 for both HOPG ( e ) and MoS 2 ( f ). Full size image The maximum value of γ lg cos θ c for the tested solvent mixtures are found to be ~24 mJ m −2 for both graphite and MoS 2 and are clustered around a surface tension of 30–35 mJ m −2 ( Fig. 1e,f ). In contrast, the γ lg cos θ c value for pure water is much smaller (~5 mJ m −2 ). As the maximum γ lg cos θ c indicates the most thermodynamically preferred solvent composition, we predict that the maximum exfoliation would occur for alcohol–water mixtures that have a surface tension around the maximum point of 30–35 mJ m −2 . Materials characterization In order to test our predictions, we proceeded to use the mixed solvents for the exfoliation of LMs. The powder LMs and the solvent mixtures described above were placed in small vials and exfoliated in a sonication bath. The colloidal suspension was then centrifuged to remove larger non-exfoliated materials. We used absorbance to characterize the colloid suspension concentration. Tapping mode atomic force microscopy (AFM), high-resolution transmission electron microscope (HRTEM) and electron diffraction (ED) was used to characterize the exfoliated flakes. An absorption spectrum of the exfoliated graphite shows a peak at 260 nm ( Fig. 2a ), which is consistent with reported values for graphene [12] . The peak position also indicates that there is no significant modification in structure or oxidation that is usually seen in graphene oxide samples with a shifted absorption peak around ~230 nm depending on the degree of oxidation [12] . A typical absorption spectrum of MoS 2 shows three peaks on 657, 602 and 385 nm ( Fig. 2f ). Based on the spectra, the exfoliated MoS 2 showed a band gap of~1.77 eV, consistent with previous studies [7] . 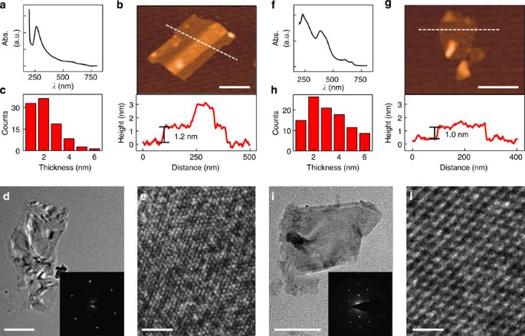Figure 2: Characterization of the exfoliated LMs. (a,f) Typical absorption spectra of the exfoliated graphene (a) with a peak absorbance at 260 nm and the exfoliated MoS2(f) with absorbance peaks at 657, 602 and 385 nm. (b,g) AFM images and section height profiles of the exfoliated graphene (b) and MoS2(g). (c,h) Sheet thickness distribution of exfoliated graphene (c) and exfoliated MoS2(h). (d,i) TEM images and ED patterns of few layer graphene (d) and MoS2(i). (e,j) HRTEM images of the exfoliated graphene (e) with a lattice spacing of 0.265 nm and MoS2(j) with a lattice spacing of 0.317 nm. Scale bars, 200 nm (b,g), 500 nm (d), 100 nm (i), 1 nm (e,j). Figure 2: Characterization of the exfoliated LMs. ( a , f ) Typical absorption spectra of the exfoliated graphene ( a ) with a peak absorbance at 260 nm and the exfoliated MoS 2 ( f ) with absorbance peaks at 657, 602 and 385 nm. ( b , g ) AFM images and section height profiles of the exfoliated graphene ( b ) and MoS 2 ( g ). ( c , h ) Sheet thickness distribution of exfoliated graphene ( c ) and exfoliated MoS 2 ( h ). ( d , i ) TEM images and ED patterns of few layer graphene ( d ) and MoS 2 ( i ). ( e , j ) HRTEM images of the exfoliated graphene ( e ) with a lattice spacing of 0.265 nm and MoS 2 ( j ) with a lattice spacing of 0.317 nm. Scale bars, 200 nm ( b , g ), 500 nm ( d ), 100 nm ( i ), 1 nm ( e , j ). Full size image AFM studies of the exfoliated graphite and MoS 2 samples on substrate show flakes with the thickness ranging from 1–6 nm are present in graphite and MoS 2 samples ( Fig. 2b,c,g,h ), indicating the presence of monolayers in the solvent, as well as few-layer materials. Scanning electron microscopy images shows both the exfoliated graphene and MoS 2 flakes have a relatively large lateral size distribution varying from 100 to 1 μm ( Supplementary Fig. S1 ). ED and HRTEM studies demonstrate that both the exfoliated graphite and MoS 2 show a hexagonal structure with lattice spacing of 0.265 and 0.317 nm ( Fig. 2d,e,i,j ) respectively, indicating no distortion in structure [15] , [16] , [17] , [18] . Together, these characterizations demonstrate that the exfoliated LMs maintain their crystalline structure during the exfoliation process with size distribution similar to previous studies, and maintain their typical crystallographic characteristics [17] , [18] . Effect of cosolvent concentration and molecular size We next investigate the effect of various solvent mixtures. We began by exploring the exfoliation rate of LMs in different water–IPA mixtures ( Fig. 3a,d ). As expected, no appreciable exfoliation was detected for both LMs in pure water due to the hydrophobic nature of the materials. Similarly, little exfoliation was observed in pure IPA after sonication. Upon mixing water with IPA in an appropriate ratio, obvious exfoliation can be observed. It appears that the exfoliation rate first increases up to a critical concentration of IPA and then decreases for both graphite and MoS 2 . Indeed, the ultraviolet-vis studies show that the exfoliation rate for both graphite and MoS 2 was not linear or monotonic with the concentration of IPA. For both graphite and MoS 2 , it appears that the exfoliation is most effective with an IPA concentration around 30 w%. Decreasing or increasing the IPA concentration could lead to a less effective exfoliation results ( Fig. 3a,d ). Photographs of the solutions of exfoliated graphene and MoS 2 also clearly demonstrate this trend ( Fig. 3b,e ). 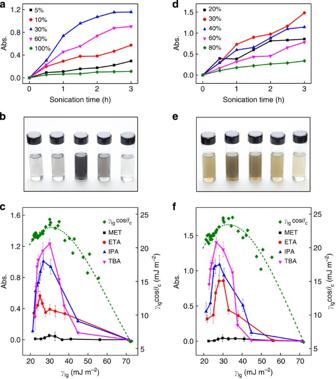Figure 3: Effect of cosolvent concentration on exfoliation. (a,d) Absorbance of exfoliated graphite (a) and MoS2(d) in various concentration of water–IPA cosolvent system as a function of sonication time. (b,e) Photographs of the exfoliated graphene in 5, 10, 30, 60, 100 w% IPA (b) and MoS2in 20, 30, 40, 60, 80 w% IPA (e) obtained after 3 h of sonication. (c,f) Absorbance of exfoliated graphene (c) and MoS2(f) in various cosolvent mixture plotted against surface tension (γlg), showing a peak around 25–30 mJ m−2for both graphite (c) and MoS2(f). The relation ofγlgcosθcversus surface tension (γlg) is also plotted in the graph with the dotted line representing a fitting curve ofγlgcosθcas a line guide to the eye. Figure 3: Effect of cosolvent concentration on exfoliation. ( a , d ) Absorbance of exfoliated graphite ( a ) and MoS 2 ( d ) in various concentration of water–IPA cosolvent system as a function of sonication time. ( b , e ) Photographs of the exfoliated graphene in 5, 10, 30, 60, 100 w% IPA ( b ) and MoS 2 in 20, 30, 40, 60, 80 w% IPA ( e ) obtained after 3 h of sonication. ( c , f ) Absorbance of exfoliated graphene ( c ) and MoS 2 ( f ) in various cosolvent mixture plotted against surface tension ( γ lg ), showing a peak around 25–30 mJ m −2 for both graphite ( c ) and MoS 2 ( f ). The relation of γ lg cos θ c versus surface tension ( γ lg ) is also plotted in the graph with the dotted line representing a fitting curve of γ lg cos θ c as a line guide to the eye. Full size image Keeping a constant sonication time of 3 h, we also compared the final concentration of exfoliated materials in MET, ETA, IPA and TBA-water mixtures. As expected from the exfoliation rate study, we saw a peak in exfoliation yield at certain cosolvent concentrations. It is noted that the alcohol concentration can vary over the 3-h sonication exfoliation process due to a solvent (alcohol) evaporation effect (see Supplementary Fig. S2 ). After correcting the solvent evaporation effect, we plotted the exfoliation yield (represented by absorbance) against the surface tension, in which a peak exfoliation yield is clearly seen at a surface tension ~25–30 mN m −2 for both graphite and MoS 2 ( Fig. 3c,f ). Cosolvent exfoliation studies on other LMs such as NbSe 2 and molybdenum trioxide (MoO 3 ) show qualitatively similar trends ( Supplementary Fig. S3 ), demonstrating the general applicability of this cosolvent approach for diverse LMs. It should also be noted that a consistent trend is observed that, at its most effective concentration, the exfoliation yield was higher for cosolvent with more –CH 3 groups for both the graphite and MoS 2 . Here we used the cosolvent molecular weight (MW of the alcohol) as a rough measure of the cosolvent molecular size due to the non-spherical shape of the molecules. When plotted against cosolvent MW, the exfoliation yield increases with increasing cosolvent MW ( Fig. 4a,b ). That is, the exfoliation yield follows the trend: MET<ETA<IPA<TBA. 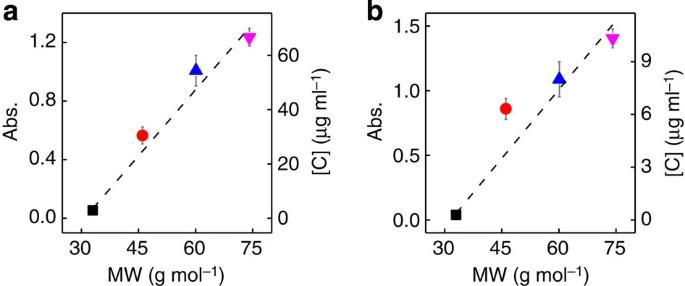Figure 4:Relationship between maximum absorbance and cosolvent MW. (a,b) Maximum absorbance of exfoliated graphene (a) and MoS2(b) plotted against cosolvent MW. Both LMs show an increased exfoliation yield for larger cosolvent molecules. Tested solvents: MET (black square), ETA (red circle), IPA (blue triangle), TBA (purple inverted triangle). Figure 4: Relationship between maximum absorbance and cosolvent MW . ( a , b ) Maximum absorbance of exfoliated graphene ( a ) and MoS 2 ( b ) plotted against cosolvent MW. Both LMs show an increased exfoliation yield for larger cosolvent molecules. Tested solvents: MET (black square), ETA (red circle), IPA (blue triangle), TBA (purple inverted triangle). Full size image The presence of maximum peak based on Young’s Equation clearly indicates that the interaction of graphite with solvent mixture is thermodynamically preferred compared with its pure water or alcohol constituents. Contact angle measurement predicts that for all tested solvents, the minimum of γ sl occurs when the solvent-mixture surface tension is around 30–35 mJ m −2 . We would like to emphasize that, as seen on Fig. 1 , the solid–liquid interaction energy ( γ sl ) is not necessarily minimized when the contact angle is zero. Contact angle is a competition between liquids at the interface whether to bond with the solid or with other liquid molecules. If the liquid–liquid interaction is weak, as measured from its surface tension, it is then more likely to form a smaller contact angle with most solid. Therefore, a smaller contact angle alone does not necessarily indicate stronger solid–liquid interaction and lower solid–liquid interface energy ( γ sl ). As expressed in the Young’s equation, the value of γ sl depends on both liquid surface tension and its contact angle with the solid surface. More generally, the equation predicts that a higher surface tension solvent with the smallest contact angle will provide higher thermodynamic stability for the liquid exfoliation of LMs. The experimental studies shows a peak exfoliation occurs at a cosolvent system with a surface tension value around 25–30 mJ m −2 for both graphite and MoS 2 ( Fig. 3c,f ), which is smaller than the predicted optimal cosolvent surface tension (~30–35 mJ m −2 ) based on the contact angle measurements and interface energy considerations ( Fig. 1e,f ). This difference can be largely attributed to the error in the contact angle measurements caused by the evaporation loss of alcohol. Owing to the relatively small liquid droplets used in the contact angle measurements and the large surface to volume ratio, this evaporation can be quite significant especially for the higher alcohol concentration solvents. Overall, this evaporation suppresses γ lg cos θ c most prominently on the higher alcohol concentration end and shifts the predicted peak exfoliation position to the right (higher surface tension values). With a correction of this evaporation effect, the predicted surface energy peak can shift left-wards to better overlap with the experimentally observed peak exfoliation position ( Supplementary Note 1 and Supplementary Fig. S4 ). The minimization of interfacial energy and observation of a peak exfoliation at certain cosolvent concentration ( Fig. 1e,f ) is somewhat counter-intuitive. It is not trivial to quantitatively explain why the interfacial energy is minimized at a certain cosolvent concentration. Qualitatively, however, the observation of the minimum interfacial energy may be explained by postulating that the cosolvent alcohol molecules behave similarly to surfactant molecules due to their tendency to aggregate in water [36] , [37] , [38] , [39] . While macroscopically alcohol mixes well with water in all proportion, microscopically the alcohol molecules can form aggregates to hide their hydrophobic group [39] , [40] , [41] , [42] . These aggregates are believed to be highly mobile and readily fluctuate. In the case of water–TBA system, these aggregates were found vary with concentration and can be as large as 40 Å (ref. 38 ). This aggregate formation is analogous to micelle formation in surfactants. The main difference of alcohols from normal surfactant is their degree of hydrophobicity. While highly hydrophobic surfactant can have critical micelle concentrations around ~1 wt%, simple alcohols require a much higher concentration (~10 s wt%) to form their aggregate. With the hypothesis that the cosolvent behaves analogously to a surfactant, we may explain the observed increase-then-decrease in the interfacial energy. Because of the hydrophobicity of the tested LMs ( Fig. 1b–d ), we believe that the alcohols acts as the main protective group that interact with surface of LMs and to prevent recombination. The non-polar -CH 3 region of the alcohol molecules is absorbed on the LM surface while its hydrophilic (-OH) group points out and interact with water to help solvate the entire system [42] . It has been shown for the case of carbon nanotubes in water-surfactant system, if the surfactant concentration is above its critical micelle concentration, the dispersion decreases [40] . The decrease in dispersion is true for most surfactant system [41] . Adding too much surfactant causes a competition between micelle formation and particle stabilization [40] , [41] . This competition reduces the effective concentration of surfactant available to protect the particle surface. By adding too much surfactant, the surfactant molecules would prefer to form micelles than being adsorbed on the particle surface. As a result, the overall dispersion decreases. This means that the most effective surfactant concentration is slightly below the critical micelle concentration, which can explain the minimum interfacial energy at certain cosolvent concentration. It would also roughly explain why more MET is needed to reach a critical concentration (less –CH 3 substituents, so less hydrophobic) compared with TBA (exfoliation peak occurs at ~80% for MET, 50% for ETA, 30% for IPA, 10% for TBA). To further confirm this hypothesis, detailed scattering experiments and molecular dynamic simulations would be necessary, which will certainly be a fundamentally interesting problem to investigate in future studies. In addition, while the contact angle measurements on HOPG predicts that the degree of exfoliation would be very similar based on the magnitude of γ lg cos θ c , our experimental results clearly show that the peak exfoliation yield differs greatly from one cosolvent mixture to another (MET<ETA<IPA<TBA). This difference suggests that there are other factors contributing to the exfoliation process in addition to the interfacial energy. As plotted on Fig. 4 , maximum exfoliation increases with cosolvent MW for both graphite and MoS 2 . The difference may be explained by the larger steric repulsion (Leonard-Jones (L-J) potential) provided by larger cosolvent molecules. Recent simulation studies suggest that the size of solvents (for example, NMP, DMF and several other solvents known to exfoliate graphite were examined) trapped in between graphene layers has an important role in the exfoliation process [42] , [43] . When two graphene sheets are separated less than a critical distance of ~6.4 Å, the L-J attraction force of the sheets dominates and expels the solvent molecules in between the sheets, favouring restack [42] , [43] . If the sheet separation is increased beyond the critical distance, the L-J attraction force between sheets is no longer significant, creating a metastable separation. It was found that the stability of the exfoliation process largely depends on steric repulsion, with some contribution by electrostatic and vdW interactions. Owing to the difficulty of expelling the trapped molecules, larger solvent molecules provide a greater steric hindrance and stabilize the separation of the graphene sheets. Experimental studies have shown consistent phenomena that the size of the trapped solvent molecules can greatly affect the recombination of mica sheets [44] . Although these studies did not explore properties of mixed solvents, we suggest that the same steric repulsion effect may be responsible for preventing recombination of both graphite and MoS 2 ( Fig. 5 ). Therefore, a larger cosolvent molecule (for example, TBA versus MET) would then provide a larger steric repulsion to promote the exfoliation. In contrast, Hansen solubility parameter does not take solvent molecule size into consideration. 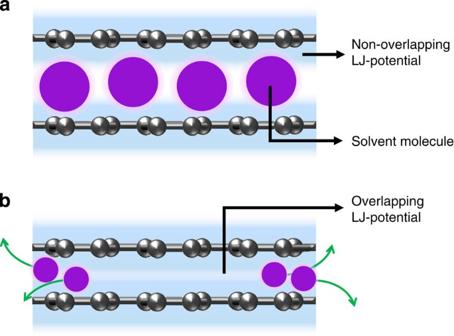Figure 5: Solvent size effect on the stability of exfoliation. (a) Large solvent molecules preventing graphene–graphene Leonard-Jones potential interaction to stabilize the inter-layer separation and exfoliation. (b) Small solvent molecules are expelled due to overlapping Leonard-Jones potential between neighbouring layers. Figure 5: Solvent size effect on the stability of exfoliation. ( a ) Large solvent molecules preventing graphene–graphene Leonard-Jones potential interaction to stabilize the inter-layer separation and exfoliation. ( b ) Small solvent molecules are expelled due to overlapping Leonard-Jones potential between neighbouring layers. Full size image We conclude that Young’s equation along with contact angle measurements can be used to evaluate the solid–liquid interfacial energy and predict the optimal exfoliation cosolvent concentration. We have shown that the interfacial energy in conjunction with steric repulsion can qualitatively predict the exfoliation efficiency of mixed solvent system. Our study provides the critical insight into the exfoliation of LMs, and defines a rational strategy for the design of an environmentally friendly pathway to high yield exfoliation of LMs. In particular, it is important to note that the addition of 10–30 w% of TBA or IPA into water can greatly increase the exfoliation yield of both graphite and MoS 2 . The low concentration of cosolvent presented here is relevant for large-scale industrial applications as the majority of our solvent is water. This reduces both the cost and many safety hazards. In addition, these solvents have a much lower boiling point compared with other commonly used liquid exfoliation solvents such as NMP (boiling point 300 °C). Processing the material after exfoliation would be easier as it is possible to evaporate the solvents through gentler heating compared with the high-boiling point solvents. Solvent mixture MET (≥99.5%), ETA (≥99.9%), IPA (≥99.5%) and TBA (≥99%) was mixed with deionized water. The surface tension of the solvent-mixture at 25 °C was obtained from CRC (refs 32 , 33 ). Contact angle measurement HOPG was purchased from nanosurf and natural single crystal MoS 2 was purchased from Wolfrm Camp Mine, Australia. These bulk LMs was used after rinsing with acetone and IPA, and vacuum dried at 100 °C. Contact angle measurement was measured at 20 °C. Data was averaged over five data points. Exfoliation Ten milligram of powder graphite (≥99%) or MoS 2 (≥99%) samples were added to a 7.5-ml glass vial. Then 5 ml of water/alcohol mixtures with weight fraction of 0 to 100 w% was added as the dispersion solvent. The samples were batch sonicated for 3 h with each sample placed in different position in the sonication bath every half-hour cycle to give uniform power distribution. In all cases, the solution was sonicated in VWR B2500A-DTH model sonication bath at high setting. The resulting dispersion was centrifuged using Eppendrof MiniSpin Plus centrifuge at 14,500 r.p.m. for 5 min. The supernatant was collected by pipette followed by another centrifugation at 14,500 r.p.m. for 15 min to further remove non-exfoliated materials. The absorbance of exfoliated graphite and MoS 2 was taken at 260 and 385 nm, respectively. Data was averaged over five independent experiments. Materials characterization Absorbance spectrum of the exfoliated materials was obtained using DU800 ultraviolet-vis spectrometer in a quartz cuvette (path length 1 cm) purchased from Starna Cell Inc. AFM samples were prepared on Si substrate. A solution of exfoliated LMs was mixed with IPA and 1-butanol, which was then added drop wise onto a distilled water surface. Free-standing film of dispersed exfoliated LMs on water surface was then scooped onto the Si-wafer surface. TEM studies were carried out on an FEI CM120 transmission electron microscope operating at 120 kV. HRTEM images were taken on an FEI Titan transmission electron microscope operating at 300 kV. How to cite this article: Halim, U. et al. A rational design of cosolvent exfoliation of LMs by directly probing liquid–solid interaction. Nat. Commun. 4:2213 doi: 10.1038/ncomms3213 (2013).